Helical nanofilaments of bent-core liquid crystals with a second twist The B4 phase of bent-core liquid crystals has been shown to be an assembly of twisted layers stacked to form helical nanofilaments. Interestingly, some of them have structural colours that cannot be explained by the nanofilaments alone. Here cryogenic-transmission electron microscopy observations on 40–120 nm films of four bent-core liquid crystal materials show that the filaments are present even in contact with a carbon substrate with only minor deformation, thus representing bulk properties. We find that the subsequent arrays of nanofilaments are not parallel to each other, but rotate by an angle of 35–40° with respect to each other. This doubly twisted structure can explain the structural colour. Being principally different from the packing of molecules in the twist grain boundary and blue phases, the double-twist structure of helical nanofilaments expands the rich word of nanostructured organic materials. The study of bent-core liquid crystals revealed many interesting and unique phenomena, including the interplay among chirality, molecular bend and director tilt [1] leading to peculiar layered structures labelled originally as B s (s=1–7) [2] , [3] , [4] . Remarkably, the B7 and B4 structures are helical in the micrometre [5] or nanometre [6] ranges, respectively. Freeze-fracture transmission electron microscopy (FFTEM) studies of the B4 phase revealed an assembly of twisted layers stacked to form chiral nanobundles with around w ~40 nm widths and h ~100 nm half pitch [6] . This helical nanofilament (HNF) phase is particularly interesting owing to its unique hierarchical nanostructure [7] , [8] in which the individual filaments further self-organize into oriented arrays of filaments that are phase coherent with respect to their twist. The bulk HNF phase expels most guest molecules, such as rod-shaped liquid crystals [9] , [10] , [11] , [12] , [13] , [14] , [15] , and their unique structure makes it attractive for the design of bulk and surface structures with controlled porosity and roughness at the nanometre and micrometre scales. For example, Kim et al . [16] demonstrated a potential application of textured HNF surfaces as self-assembled super hydrophobic layers. Other applications are envisioned in nonlinear optics, chiral separations and photovoltaics. Solar cells require thin films in the range of hundred nanometres, so it is desirable to know the structure of the HNF phase in such thin films. Recent FFTEM studies, for example, showed the formation of focal conic structures instead of the helical nanofilaments near a glass substrate [17] , which indicates that the structure near a surface can be different from the bulk structure. While FFTEM monitors the profile of a broken surface of a bulk (over micrometre thick) material, cryo-transmission electron microscopy (TEM) gives information about the inside of a thin (L~100 nm film) material; therefore, it can provide complementary information of the structures. Indeed, it was shown recently that cryo-TEM is suitable to visualize smectic layers of thermotropic liquid crystals [18] . In this paper we describe cryo-TEM studies of the phenylene bis(alkoxyphenyliminomethyl) benzoate series [8] , [19] with n =7, 8, 9 and 12 that form room temperature HNF phases. The most important result of the study is that the nanofilament layers stack on top of each other in a twisted configuration; the carbon substrate has only minor effect on the bulk structure of the helical nanofilaments. The HNF phase thus features a double twist: one axis of twist is defined along the axis of each nanofilament; the orthogonal second axis of twist describes the rotation of the nanofilament layers. This double twisted structure explains the peculiar bulk optical properties of HNF phases, such as colour and optical activity. Optical spectra and small angle X-ray measurements The studied phenylene bis(alkoxyphenyliminomethyl) benzoate series [8] , [19] with n =7, 8, 9 and 12 carbons in their alkyloxy tails were synthesized by D Lötzsch in G Heppke’s group at the Iwan Stranski Institute of the Technical University, Berlin, Germany. Their molecular structures, phase sequences, colour images with the corresponding reflection spectra and the small angle X-ray scattering (SAXS) results are shown in Fig. 1 . 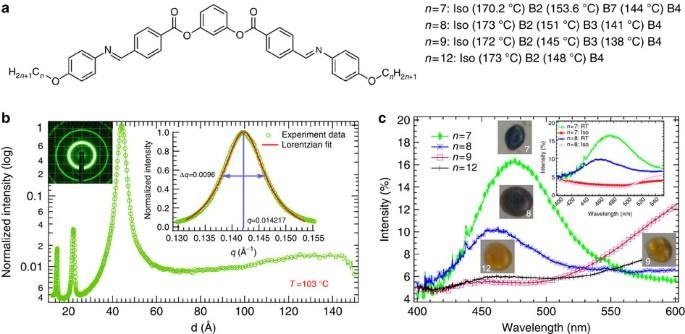Figure 1: Characterization of phenylene bis(alkoxyphenyliminomethyl) benzoate (PnOPIMB). (a) Molecular structure and phase sequence of PnOPIMB (n=7, 8, 9 and 12) in cooling at 1 °C min−1. (b) SAXS intensity ind-space for P7OPIMB at 103 °C. The inset on the left shows the two-dimensional diffraction pattern, and the right inset illustrates theq-dependence of the normalized intensity around the strongest peak. (c) Optical appearance of the materials in bulk. Main panel shows the reflection spectra and the corresponding colour images of drops at room temperature. The inset compares the spectra of P7OPIMB and P8OPIMB at room temperature and the isotropic phase, indicating that the blue reflection is related to the B4 structure of the materials. Figure 1b shows the length dependence of the normalized SAXS intensity for P7OPIMB at 103 °C. The main peak occurs at d =44 Å with two clearly visible higher harmonics showing well-defined layering. No other periodicity up to 15 nm length scales can be found. The correlation length ξ =2/Δ q =21 nm corresponding to a domain size w~ 2, ξ ~40 nm (Francescangeli et al . [20] ), is in accordance with the typical width of the helical nanofilaments found by FFTEM [6] . Polarizing optical microscopy textures of 5–10 μm films are grainy dark blue indicating low birefringence in the B4 phase. Uncrossing the analyser by ±10° reveals large (up to 1 mm size) interchanging darker and lighter domains, revealing optical activities with opposite signs. In non-polarized white light the homologues with n =7 and 8 have dark opal colour in the entire HNF phase with reflection peaks at 475 nm and 460 nm, respectively, whereas the n =9 and 12 homologues are yellow (see Fig. 1c ), and their reflected intensities have only minor peaks at around 450 nm. Importantly, the low wavelength peaks of P7OPIMB and P8OPIMB disappear in the B3, B2 and isotropic phases (see inset of Fig. 1c ) and they also become yellow, related to the absorption of the Schiff base in the molecules. The blue appearance of the lower homologues was noted in a previous work [8] (and attributed to a helix along the smectic layers), but the absence of the blue reflection in the higher homologues has never been discussed. Figure 1: Characterization of phenylene bis(alkoxyphenyliminomethyl) benzoate (PnOPIMB). ( a ) Molecular structure and phase sequence of PnOPIMB ( n =7, 8, 9 and 12) in cooling at 1 °C min −1 . ( b ) SAXS intensity in d -space for P7OPIMB at 103 °C. The inset on the left shows the two-dimensional diffraction pattern, and the right inset illustrates the q -dependence of the normalized intensity around the strongest peak. ( c ) Optical appearance of the materials in bulk. Main panel shows the reflection spectra and the corresponding colour images of drops at room temperature. The inset compares the spectra of P7OPIMB and P8OPIMB at room temperature and the isotropic phase, indicating that the blue reflection is related to the B4 structure of the materials. 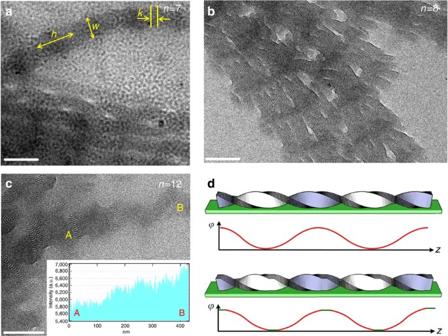Figure 2: TEM images and model structures of individual helical nanofilaments. (a–c) Cryo-TEM images showing the growing of individual nanofilaments in phenylene bis(alkoxyphenyliminomethyl) benzoate withn=7, 8 and 12. Insert incshows the variation of the transmitted electron intensity from A to B. The larger intensity at B indicates thinner material. (d) Model structures and the variation of the angleϕdefined as the angle between the substrate and the smectic layer normal. Top part illustrates the non-deformed HNF observed in bulk and the bottom shows the proposed structure on a substrate. Scale bars, 100 nm (a–c). Full size image Cryo-TEM measurements Figure 2a–c shows the cryo-TEM images of the individual helical nanofilaments for the homologues n =7, 8 and 12, respectively. Their average thickness appears to be about 40 nm, which is in agreement with previous FFTEM results, although they are getting thinner towards the tip of the filaments. This is illustrated in the inset of Fig. 2c , which shows that the transmitted electron intensity measured along the helical axis increases (indicating decrease of the thickness) towards the tip. The TEM textures show families of parallel fringes of an approximate extension k ~10±4 nm along the filament axis that appear periodically along the filaments with a period h ( Fig. 2a ) that varies in the short range 100–120 nm from one homologue to another. The period h of the families of fringes equals half pitch of the nanofilaments found in FFTEM experiments by Hough et al . [6] , indicating that the filaments in Fig. 2 grow parallel to the substrate. The separation d between the fringes within the same family is much smaller than h and corresponds to the smectic layer spacing obtained from SAXS measurements. This indicates that the fringes mark the regions in which the smectic layers are close to the upright orientation with respect to the substrate. The contrast of fringes is provided by the electron density difference between the aromatic cores and hydrocarbon tails [18] . The parameters h and d for different homologues do not vary much: n =7: h =118±3 nm and d =4.48 nm; n =8: h =130±3 nm and d =4.60 nm; n =9: h =122±3 nm and d =4.87 nm; n =12: h =107±3 nm and d =4.64 nm. Interestingly, the contrast of fringes is nearly constant over their extension k , which is not fully compatible with the model of continuously twisting and bending helical nanofilaments. Figure 2: TEM images and model structures of individual helical nanofilaments. ( a – c ) Cryo-TEM images showing the growing of individual nanofilaments in phenylene bis(alkoxyphenyliminomethyl) benzoate with n =7, 8 and 12. Insert in c shows the variation of the transmitted electron intensity from A to B. The larger intensity at B indicates thinner material. ( d ) Model structures and the variation of the angle ϕ defined as the angle between the substrate and the smectic layer normal. Top part illustrates the non-deformed HNF observed in bulk and the bottom shows the proposed structure on a substrate. Scale bars, 100 nm ( a – c ). Full size image The layer positions of an ideal HNF running along z can be given [21] by the equations: x = w cos ϕ ; y = d +sin ϕ and ϕ =π· z / h (see upper part of Fig. 2d ). With parameters w ~40 nm , h~ 100 nm and d ~5 nm, we obtain that the contrast should completely disappear within a 3-nm distance from the inflection point, so that one would expect to see only dots centred in fan (or hour glass)-shaped domains with fading contrast. One might suggest that this nearly constant contrast of fringes could be a result of a twist grain boundary (TGB)-like structure where the layers are broken into blocks of thickness k ~10 nm that rotate around z in ~10° steps. However, a bulk TGB-like structure with such periodic blocks would result in a peak in the SAXS profile at ~10 nm, which was not observed (see Fig. 1b where the scattering intensity is almost constant in the 6–14-nm range). For this reason we propose that the structure is essentially a helical nanofilament with a small deformation induced by surface adhesion of molecules in ‘tangential’ orientation, which explains a tendency of smectic layers to remain perpendicular to the bounding surface within a finite interval close to the observed value of k . Such an HNF is flattened around the ϕ =0, ±π, ±2π,...positions (see lower part of Fig. 2d ), but since the extension k of the flattened region is much smaller than the half pitch h of the nanofilament, the overall modification of the ideal HNF shown in the upper part of Fig. 2d is insignificant. Therefore, we conclude that even the first layer is made of helical filaments. This is very different from prior FFTEM studies on the n =7 homologue near a flat and rigid glass substrate that revealed focal conic domains formed under the influence of the surface forces near the substrate [17] , [22] . Our observations of only slightly distorted nanofilaments suggest that the carbon substrate preserves the structural features pertinent to the bulk structure of the HNF phase, despite the relatively small thickness of the samples (40–120 nm). Overall, the TEM textures of helical filaments in Fig. 2 are very similar to the TEM textures of rods formed by mesoporous silica with helical twist [23] , [24] , [25] , [26] . An interesting feature of both systems is that the families of parallel fringes can be bent. The bending is especially evident for n =9 and n =12; in the homologues with n =7 and n =8, the fringes are relatively straight ( Fig. 2a–c ). The bend of fringes correlates with the bend of the contour of the entire filament. As demonstrated in Figure 5 of Che et al . [23] , the bent fringes result from a tilted orientation of the rods, that is, the bend is observed when the axis of the rods is not strictly perpendicular to the electron beam. Our observation of the bent fringes suggests that the axes of helical nanofilaments might not be always strictly parallel to the substrates. This tilting effect can be caused by a simple tilt of the sample in the TEM chamber, or by the conditions of filament directional growth. If one end of the filament is thicker than another, the tilt of the axis is inevitable. 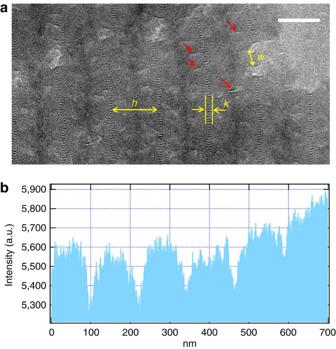Figure 3: Cryo-TEM image and intensity profile of P9OPIMB. (a) TEM image of fused parallel filaments in a P9OPIMB sample quenched at 55 °C. Short (k~10 nm) stripes separated by the layer spacingd~4.64 nm appear periodically with half pitchh=120 nm along the filament. Red arrows point to elongated scars due to partial voids. Scale bar, 100 nm. (b) Transmitted electron intensity along the periodicity with half pitchh. Figure 3a shows an area of fully developed and fused parallel arrays of one layer of filaments running parallel to the substrate. The fringes of extension k are running parallel (nearly vertical in the picture) to each other, and it is difficult to see the borderline between the individual filaments. This is somewhat surprising because from the shape of the individual filaments one would expect voids for certain phases of twist between two adjacent filaments. Although we see some lighter elongated scars (see also on Fig. 4 ) running along the stripes owing to defects or partial voids, the individual filaments should definitely change shape to fill out that space as well. Remarkably, this is done so that the parameters h and k found in the individual filaments remain unchanged. Figure 3: Cryo-TEM image and intensity profile of P9OPIMB. ( a ) TEM image of fused parallel filaments in a P9OPIMB sample quenched at 55 °C. Short ( k ~10 nm) stripes separated by the layer spacing d ~4.64 nm appear periodically with half pitch h =120 nm along the filament. Red arrows point to elongated scars due to partial voids. Scale bar, 100 nm. ( b ) Transmitted electron intensity along the periodicity with half pitch h . 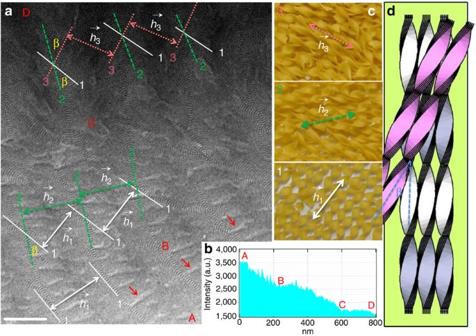Figure 4: TEM image and models showing double-twist structure. (a) Cryo-TEM image of an area of P8OPIMB with gradually increasing thickness from right bottom to left top. The vectors,andillustrate the direction and periodicity of the filaments. Scale bar, 100 nm. (b) Transmitted electron intensity profile along the line ABCD, indicating a gradual increase of the film thickness from A to D. (c) Equilibrium arrangement of different layers of helical pastas; from bottom to top is the first, second and third layer of filaments, respectively. (d) Sketch of the proposed arrangement of the helical nanofilaments. Full size image Figure 4: TEM image and models showing double-twist structure. ( a ) Cryo-TEM image of an area of P8OPIMB with gradually increasing thickness from right bottom to left top. The vectors, and illustrate the direction and periodicity of the filaments. Scale bar, 100 nm. ( b ) Transmitted electron intensity profile along the line ABCD, indicating a gradual increase of the film thickness from A to D. ( c ) Equilibrium arrangement of different layers of helical pastas; from bottom to top is the first, second and third layer of filaments, respectively. ( d ) Sketch of the proposed arrangement of the helical nanofilaments. Full size image Figure 3b illustrates the variation of the transmitted intensity along the periodicity with half pitch h . We can see a periodic variation so that the intensity is smallest (the picture is darkest) exactly in between the stripes. This may indicate that the thickness of a filament is largest in the area where the layers are parallel to the substrates. However, this does not correspond to the ideal HNF or the surface-deformed HNF model shown in Fig. 2d , indicating that the transmitted electron intensity depends on the orientation of the layers. This is also unexpected, as the total length of the core and tail areas an electron needs to pass through is independent of the angle, provided that the layers deviate from the vertical direction by more than α =tan −1 ( d/L )~tan −1 ( d/w )~6°. More studies and mathematical modelling are needed to clarify this issue. Figure 4a illustrates an area of P8OPIMB with decreasing transmitted electron intensity, indicating increasing film thickness from the bottom to the top of the picture. At the bottom (area A) of the picture we can see the parallel stripes appearing periodically along a direction labelled similar to the texture of one layer of parallel array of filaments shown in Fig. 3 . In this picture the white scars indicating the interface between adjacent filaments are more pronounced, and they show an overall splay of the filament array. As the film thickness increases from B to C, a splitting of the stripes by about β=30–40° can be observed. The second direction ( ) of the stripes can be interpreted as a result of a second layer with filaments’ direction rotated with respect to first layer by an angle β. A third set of stripes appears between C and D with orientation along , rotated by angle β with respect to . The transmitted electron intensity measured along a line defined by A, B, C and D (see inset in the right-bottom corner) shows decreasing values with some plateaus at A, B and C. The difference between the intensities in the plateaus is roughly the same (about 900), marking the thickness of one layer of filaments (~40 nm). Similar trends were observed for n =7, and in small areas even for n =9 and 12 homologues. These observations can be interpreted as overlapping HNFs where the filaments of the subsequent layers are rotated by β~30–40° with respect to each other. Interestingly, Chen et al . [17] have already observed that at the surfaces, where parabolic domain walls form, the HNFs axes are tilted by γ~38° with respect to a periodic one-dimensional modulation. However, this rotation was not explained, and no subsequent rotations of the filaments with respect to each other was assumed [22] . On the basis of similarity of these two angles (γ and β), we propose they have the same geometrical origin. The directions of the smectic layers of a helical nanofilament are different at the bottom and the top (see top of Fig. 2d ), as they make an angle θ=±tan −1 ( w/h ) with respect to the helical axis. For w =40 nm and h =120 nm, θ=18.4°, that is, the difference between the angles on opposite sides is 2θ~37°, corresponding to β of Fig. 2d . To show that the rotation of the filaments has a geometrical mechanism (close packing), we carried out a simple experiment by using commercially available twisted noodles having shape similar to our model nanofilaments. This experiment is illustrated in Fig. 4c . First, we glued about 150 noodles aligned uniformly in horizontal direction to the bottom of a rectangular pan (see bottom of Fig. 4c ); then we added 150 noodles randomly on the top of the aligned layers and vertically vibrated the pan with a speaker at frequency f =40–70 Hz with acceleration of ~1 m s −2 for half an hour until a steady configuration of the noodles formed. As seen in the middle picture of Fig. 4c , the average direction of the second layer is rotated by about 40° with respect to the first one. Finally, we added an additional 150 noodles on the top of the second layer and vibrated the pan again for an additional half hour. As shown in the top picture of Fig. 4c , the resulting configuration of the third layer is also fairly uniform, but now rotated by about 80° with respect to the first layer. Although the helical nanofilaments grow via nucleation, their direction can be also adjusted by thermal motion; thus, this simple experiment can be demonstrative. Motivated by this similarity, we propose that the packing of the subsequent layers of helical nanofilaments is as illustrated in Fig. 4d . In this model, smectic layers near the interface of adjacent filaments have the same orientation, which means that the axes of filaments are rotated with respect to each other by an angle β~37°. Finally, we propose that the rotation of the subsequent arrays of filaments can explain the blue reflection colour observed in the n =7 and 8 homologues with straight filament axes (see Fig. 1c ). Taking the narrowest thickness of the individual filaments ~30 nm and the rotation angle β~37°, a full rotation takes about 10 layers, that is, about 300 nm length. Multiplying this with the refractive index of n o ~1.6, we can explain the selective reflection at about λ ο ~480 nm seen in Fig. 1c for the n =7 and 8 homologues. This peak is very weak in the n =9 and 12 homologues, apparently because the individual filaments grow in a tilted manner and result in a less regular packing, which does not allow long-range synchronizations of the secondary twist; the issue needs to be studied further. The doubly twisted structure of the HNF phase resembles the TGB phase in that there are blocks and finite rotation angles; however, in the HNF the blocks are not straight layers, but continuously twisting filaments. The double twist of the nanofilaments is also different from the double twist observed in various types of blue phases of either cholesteric [27] or smectic [28] nature. The blue phases are made of chiral molecules that pack into doubly twisted cylinders with a single periodicity and only one sense of chirality determined by the molecular chirality. In contrast, the HNF phase has ambidextrous chirality because the molecules are non-chiral. This can explain the ambidextrous optical activity observed in the HNF phase by polarizing optical microscopy. In addition, they have two different periodicities: one associated with the continuous twist of the individual filaments (~200 nm) and the other with a gradually twisted packing (~300 nm). We note that in the bulk there is no substrate to direct the orientation of the first layer of filaments and there should be microscopic domains with different secondary twist direction. To summarize, we demonstrate a new architecture of the helical nanofilaments in thin (40–120 nm) films of four bent-core materials. Our results show that the HNF phase in thin films comprises twisted layers of nanofilaments, yielding a double twisted structure of the bulk arrangements of the nanofilaments. The new insight is made possible by the cryo-TEM observation technique that probes the transmitted intensity of the electron beam passing through the bulk of the sample and thus yields three-dimensional structural information. Such an insight is not readily available with the traditionally used FFTEM approach, in which one observes only the fractured surface with essentially two-dimensional features. The double-twist structure can explain the mysterious properties of the HNF materials, such as structural colour and ambidextrous optical activity. Being principally different from the packing of molecules in other twisted structures, the double-twist structure of HNF expands the rich word of nanostructured organic materials, giving structural colours to various living creatures, or utilized in photonic band gap materials. In spite of the clear new features presented here, there remain a number of unexplained features such as the curved shape of the filaments and the variations in the intensity profiles of the TEM images. Small angle X-ray measurements SAXS measurements were performed at the National Synchrotron Light Source (beam line X6B) of Brookhaven National Lab. The materials were filled into 1 mm diameter quartz X-ray capillary tubes, which were then mounted into a custom-built aluminium cassette that allowed X-ray detection with ±13.5° angular range. The cassette fits into a standard hot stage (Instec model HCS402) that allowed temperature control with ±0.1 °C precision. The stage also included two cylindrical neodymium iron boron magnets that supplied a magnetic induction of B =1.5 T perpendicular to the incident X-ray beam. Two-dimensional SAXS images were recorded on a Princeton Instruments 2084 × 2084 pixel array charge-coupled device detector. The beamline was configured for a collimated beam (0.2 × 0.3 mm 2 ) at energy 16 keV (0.775 Å). Details of the experimental conditions are described elsewhere [29] . Cryo-TEM The cryo-TEM measurements were carried out on a FEI Tecnai F20 microscope, operating at 200 kV and equipped with a Schottky field emission gun and a twin-blade anti-contaminator. The microscope provides 0.24 nm point-to-point resolutions and a 0.15-nm information limit in TEM mode. A Gatan cryoholder (model 626.DH) made it possible to keep the specimen temperature below −170 °C throughout the TEM observation. All images were recorded using a Gatan 4 K Ultra Scan charge-coupled device camera. As liquid crystal films are sensitive to the electron beam irradiation, the films were normally previewed rapidly at a dose of 20 e − nm −2 . Selected areas were then imaged at a dose level of 200 e − nm −2 , which we found did not cause any radiation damage. Previous studies on ~100 nm thermotropic bent-core liquid crystals films carried out with this instrument demonstrated the possibility to visualize smectic layers with a resolution better than 0.7 nm (Zhang et al . [18] ) In contrast to FFTEM, which visualizes the topography of a replica in form of bright and shadowed areas with 2–3 nm resolution, cryo-TEM reveals a periodicity of layers when they are nearly parallel to the electron beam. How to cite this article: Zhang, C. et al . Helical nanofilaments of bent-core liquid crystals with a second twist. Nat. Commun. 5:3302 doi: 10.1038/ncomms4302 (2014).